Broadband polarization-independent resonant light absorption using ultrathin plasmonic super absorbers Resonant plasmonic and metamaterial structures allow for control of fundamental optical processes such as absorption, emission and refraction at the nanoscale. Considerable recent research has focused on energy absorption processes, and plasmonic nanostructures have been shown to enhance the performance of photovoltaic and thermophotovoltaic cells. Although reducing metallic losses is a widely sought goal in nanophotonics, the design of nanostructured 'black' super absorbers from materials comprising only lossless dielectric materials and highly reflective noble metals represents a new research direction. Here we demonstrate an ultrathin (260 nm) plasmonic super absorber consisting of a metal–insulator–metal stack with a nanostructured top silver film composed of crossed trapezoidal arrays. Our super absorber yields broadband and polarization-independent resonant light absorption over the entire visible spectrum (400–700 nm) with an average measured absorption of 0.71 and simulated absorption of 0.85. Proposed nanostructured absorbers open a path to realize ultrathin black metamaterials based on resonant absorption. Noble metals such as silver, gold and copper are excellent reflectors at infrared and lower frequencies, but exhibit plasmon resonances at visible frequencies. By structuring noble metal surfaces on the subwavelength scale, localized and delocalized surface plasmon resonances can be designed to produce high absorption on otherwise reflective surfaces. Resonant light absorption in metallic structures has been widely studied both theoretically and experimentally in arrays of metallic gratings [1] , [2] , [3] , [4] , [5] , nanoparticles [6] , [7] and subwavelength slits [8] , [9] . Metamaterials are also promising candidates to enhance electromagnetic wave absorption, and have been shown to yield perfect absorption at microwave [10] , terahertz [11] and infrared [12] , [13] , [14] frequencies. To date, however, resonant absorption schemes using plasmonic nanostructures and metamaterials have been designed to absorb light within a narrow wavelength range, and with few exceptions [6] , [7] , [14] , the resonant absorption behaviour strongly depends on the incident polarization. Achieving a resonant response that spans a broad wavelength range is required for broadband thin-film thermal emitters [15] , and thermophotovoltaic [12] cells, as well as plasmonic scatterers [16] , [17] , [18] for photovoltaic cells. Recently, Pendry and collaborators [19] outlined a theoretical framework based on conformal mapping transformations to design plasmonic nanostructures that have a large absorption cross-section over a broad range of frequencies. Using a transformation optics design approach, Narimanov and Kildishev [20] have proposed optical black holes that are capable of absorbing light over a large frequency range. While there is great interest in achieving 'black' materials exhibiting large broadband absorption using plasmonic and metamaterial designs, this concept cannot be straightforwardly realized using conventional plasmonic motifs such as metallic nanoparticle and nanoscale gratings, due to the inherently narrow-band plasmon resonances associated with these structures. Here, we propose and demonstrate experimentally realizable ultrathin planar plasmonic super absorbers that are capable of absorbing light from 400 nm to 700 nm with a measured average absorption of 71%. Moreover, the absorption is independent of the incident polarization due to the symmetric arrangement of crossed trapezoid array geometry utilized in the absorber design. Our metallo-dielectric absorber is a clear departure from black materials formed from optically thick, micro-structured materials that are absorbers in bulk form, such as semiconductors [21] , [22] and carbon nanotubes [23] , [24] , [25] , and employs a structure of subwavelength thickness whose constituent materials are lossless dielectrics and highly reflective metals. Nanostructured metal–insulator–metal absorber structures Our broadband absorber consists of a three-layer metal–insulator–metal (MIM) thin-film laminate where only the top metal layer is patterned. Two examples of such thin-film MIM absorbers are metal stripe ( Fig. 1a ) and trapezoid arrays ( Fig. 1b ) that are periodically arranged along the x axis with a periodicity of 300 nm. The top and bottom Ag layers of the MIM stack are 100 nm thick, and the middle SiO 2 layer thickness is 60 nm. The thicknesses of these layers are the same for all of the MIM absorber structures reported in this article. Metal stripes of two different widths, w =60 nm and w =120 nm, with a periodicity of 300 nm were fabricated using electron beam (e-beam) lithography. 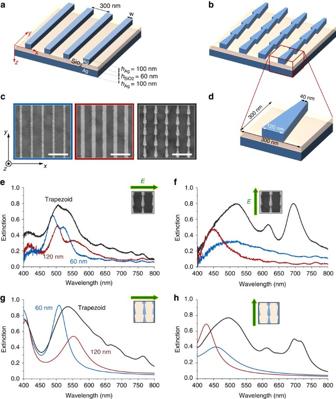Figure 1: Polarization-dependent light absorbers based on metallic gratings and trapezoid arrays. (a) Schematic representation of a three-layer MIM system with the top layer patterned as metallic gratings of widthw. (b) Schematic representation of trapezoid array. (c) SEM images of metallic gratings withw=60 and 120 nm, and trapezoid arrays. Scale bar is 500 nm. (d) Schematic representation of the unit cell of a single trapezoid, width varying from 40 nm to 120 nm over 300 nm. (e) Measured extinction spectrum for the 60 nm and 120 nm wire gratings and trapezoid arrays for TM polarization (inset). (f) Measured extinction spectrum for TE polarization (inset). (g,h) Simulated extinction spectrum for TM and TE polarizations. Scanning electron microscopy (SEM) images of the fabricated structures are shown in Figure 1c . Figure 1d depicts a schematic drawing of such a metallic trapezoid unit cell that is periodic along the x and y axes with a periodicity of 300 nm ( Fig. 1b ). Figure 1: Polarization-dependent light absorbers based on metallic gratings and trapezoid arrays. ( a ) Schematic representation of a three-layer MIM system with the top layer patterned as metallic gratings of width w . ( b ) Schematic representation of trapezoid array. ( c ) SEM images of metallic gratings with w =60 and 120 nm, and trapezoid arrays. Scale bar is 500 nm. ( d ) Schematic representation of the unit cell of a single trapezoid, width varying from 40 nm to 120 nm over 300 nm. ( e ) Measured extinction spectrum for the 60 nm and 120 nm wire gratings and trapezoid arrays for TM polarization (inset). ( f ) Measured extinction spectrum for TE polarization (inset). ( g , h ) Simulated extinction spectrum for TM and TE polarizations. Full size image Polarization-dependent absorption in metallic stripe arrays Total transmission ( T ) and reflection ( R ) from the MIM absorbers are measured using an inverted optical microscope, and extinction is defined by 1- T - R . The use of an optically thick 100 nm Ag back-reflector, the bottom layer of the MIM stack, prevents light transmission and reduces the extinction to 1- R . Optical measurements are performed at normal incidence for two different polarizations, electric field perpendicular (TM) and parallel (TE) to the wire axis ( y axis). Figure 1e plots the measured extinction spectra of the 60 nm (blue line) and 120-nm-wide (red line) metallic stripe arrays excited with TM polarization. Localized surface plasmon resonances can be identified from the extinction peaks in the spectra, and they typically yield narrow-band resonances depending on the width of the metal wire. As expected, the localized surface plasmon resonance redshifts with increased wire width. For the 60-nm-wide metallic stripe array, the resonance peak is observed at 488 nm with the maximum extinction value of 0.65, whereas for the 120-nm-wide stripe the maximum extinction is 0.51 measured at 507 nm. The presence of both the dielectric and metal films underneath the nanostructured layer results in a hybridized mode due to the coupling of the metal stripes with the planar Ag film [4] . Under TE polarization, where the E-field is parallel to the wires, the wire arrays behave as an effective plasma media [26] . Different widths result in different effective plasma frequencies as seen in Figure 1f ; however, the extinction is not as strong as for the case of TM polarization. Clearly, the resonant absorption behaviour depends on the incident polarization for the metallic stripe arrays. Recently, metallic wire arrays have been theoretically shown to enhance light absorption in silicon thin-film solar cells [18] . By designing a broader and polarization-independent light harvesting structure, the performance of such plasmonic photovoltaic devices could significantly be improved. Trapezoid arrays for broadband resonant absorption The optical absorption of MIM gratings occurs over a rather narrow wavelength regime, but we find metallic arrays of trapezoids ( Fig. 1b ) access a broader wavelength optical response. An SEM image of the fabricated trapezoid array is shown in the right panel of Figure 1c . Under TM polarization ( Fig. 1e inset), a broader and higher extinction peak is observed from the trapezoid array compared with the metal stripe array. A different transverse resonance is excited at each width along the trapezoid. Broadband extinction for TM polarization arises from the resonant electromagnetic responses of different cross-sections of the trapezoid at different wavelengths. The maximum extinction is measured to be 0.77 at 504 nm. Under TE polarization, we observe enhanced extinction over the entire visible spectrum in the trapezoid arrays ( Fig. 1f ). A resonance is excited around 720 nm, which is attributed to the longitudinal dipole resonance of each trapezoid (300 nm) whose long axis is parallel to the incident electric field. Although individual trapezoids are concatenated into contiguous arrays, the longitudinal dipole resonances of each trapezoid are observed. Moreover, the discontinuities at the junctions between short and long sides of adjacent trapezoids allow the excitation of broad localized resonances at shorter wavelengths. However, in both the linear metal stripe and metal trapezoid arrays, resonant light absorption is strongly dependent on the polarization of the incident light. We also performed full-field electromagnetic simulations of linear metal stripes and trapezoid arrays, and the corresponding results for TM and TE polarization are plotted in Figure 1g,h, respectively. The finite-difference time-domain (FDTD) simulations utilized metallic shapes that were obtained from digitized SEM images of a 2×2 unit cell of experimentally fabricated trapezoid arrays, as shown in the insets of Figure 1g,h . Overall, we obtained remarkably good agreement between the experiments and simulations in terms of predicting the resonant peak positions in the extinction spectrum. Moreover, we have performed the finite difference frequency domain (FDFD) simulations for metallic stripes only as plotted in Supplementary Figure S1 . FDTD and FDFD simulations provided comparable results assuring that the broadband source excitation in FDTD will not be an issue. We noticed that the extinction values in the experiments are in general lower than the simulated values. In the simulations, the extinction is calculated in the near-field of the absorbers for the normal incident light. However, in the experiments, extinction is measured in the far-field over a finite acceptance angle within the light cone. Additionally, the fabricated samples have rougher surfaces than the metal films assumed in the simulations, and experimental surface roughness may cause additional scattered light to be collected within the light cone. To gain insight on the localized surface plasmon resonance and the effect of trapezoid shape in broadening the extinction spectra, we calculated the magnetic field profiles for TM-polarized ( E // x ) excitation. The magnetic field intensity for the w =120-nm-wide metallic stripe array in the x–z plane (as shown with red plane in Fig. 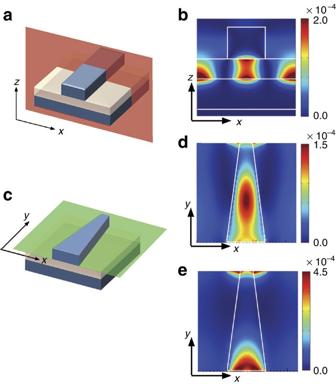Figure 2: Magnetic field profile at the localized surface plasmon resonance frequency. (a) Three-dimensional schematic view of 120-nm metallic grating showing the cross-section alongx–zplane (red plane). (b) Calculated magnetic field intensity for 120 nm stripe at 555 nm on thex–zplane as shown inFigure 2a. (c) Three-dimensional schematic view of single trapezoid unit cell showing the cross-section alongx–yplane at the top Ag/bottom SiO2interface (green plane). (d) Calculated magnetic field profiles in thex-yplane for single trapezoid unit cell as shown inFigure 2catλ=515 nm and (e) atλ=555 nm. 2a ) is plotted in Figure 2b . The magnetic field at λ =555 nm (the reflection peak of 120 nm stripes) is strongly localized in the dielectric region between the top and bottom metallic layers. For the trapezoid array simulations, we employed an idealized trapezoid single unit cell with periodic boundary conditions along x - and y -axes. We calculated the magnetic and electric fields intensities at two different wavelengths (515 and 555 nm) in the top Ag metallic trapezoid–dielectric layer interface, as shown with green plane in Figure 2c . Magnetic field intensities are plotted in Figure 2d,e for λ =515 nm and λ =555 nm, respectively. At 515 nm, the magnetic field is stronger in the middle section of the trapezoid unit cell. However, at 555 nm, the magnetic field intensity is strongly localized at the widest edge of the trapezoid. Figure 2: Magnetic field profile at the localized surface plasmon resonance frequency. ( a ) Three-dimensional schematic view of 120-nm metallic grating showing the cross-section along x–z plane (red plane). ( b ) Calculated magnetic field intensity for 120 nm stripe at 555 nm on the x – z plane as shown in Figure 2a . ( c ) Three-dimensional schematic view of single trapezoid unit cell showing the cross-section along x–y plane at the top Ag/bottom SiO 2 interface (green plane). ( d ) Calculated magnetic field profiles in the x - y plane for single trapezoid unit cell as shown in Figure 2c at λ =515 nm and ( e ) at λ =555 nm. Full size image Polarization-independent resonant absorption in crossed trapezoidal arrays In order to achieve a polarization-independent electromagnetic response, a top metallic layer consisting of an array of crossed metallic gratings can be utilized, with the widths and periods of the crossed wires being equal [2] . Such a symmetric configuration yields the same optical responses for TM and TE polarizations. Here, we studied two different crossed gratings with the crossed wire widths of w =60 nm and w =120 nm ( Fig. 3a ). 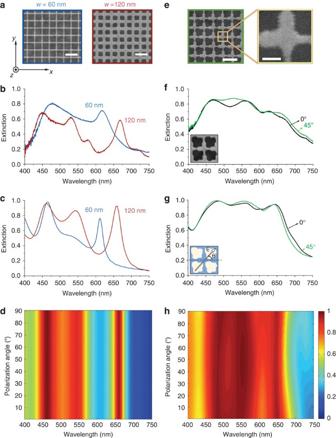Figure 3: Crossed metallic gratings and broadband, polarization-independent plasmonic super absorbers. (a) SEM images of two different crossed metallic gratings withw=60 and 120 nm. Scale bars are 500 nm (b) Measured and (c) Simulated extinction spectra for two different crossed metallic gratings. (d) Extinction spectra for 120-nm-wide crossed-grating structure as a function polarization angle and wavelength. (e) SEM image of the fabricated crossed trapezoid arrays (left) and a single unit cell of crossed trapezoid (right). Scale bars are 500 and 100 nm, respectively. (f) Measured, and (g) Simulated extinction spectra using digitized SEM images (inset) for different incident electric field polarization angles (inset). (h) Extinction spectra for crossed trapezoid array as a function polarization angle and wavelength. The measured extinction spectra of these gratings are plotted in Figure 3b . In addition to the MIM resonances at shorter wavelengths, additional localized plasmon resonances are excited at longer wavelengths due to the square nanohole arrays formed by the gap between the neighbouring stripes. For fishnet gratings of 120 nm width, four different resonant peaks are observed in the extinction spectra, at 450, 532, 578 and 668 nm, whereas for the 60-nm-wide fishnet structures the resonant peaks reduce to two distinct peaks at 477 and 617 nm. Clearly, resonant responses spanning the whole visible spectrum could potentially be obtained with different grating linewidths and periods, but in each case the extinction is not broad enough to yield resonant super absorption over the whole visible spectrum. Electromagnetic simulations are performed with ideal crossed gratings, and the results plotted in Figure 3c agree with the experimental data in terms of the spectral shapes. For the 120-nm-wide crossed gratings though, there is an additional measured peak at 578 nm that does not seem in the simulations. We attribute this peak to possible deviation of the experimentally fabricated samples from the ideal design. In order to demonstrate polarization-independent resonant light absorption with the crossed-grating geometry, we performed additional simulations with 1° increments in polarization angle for the 120-nm-wide crossed grating. Figure 3d plots the corresponding extinction spectra as a function of both polarization angle and wavelength. As seen in the figure, the extinction spectra do not depend on the incident polarization; however, one can observe slight changes such as reduced extinction around 515 nm. This is due to the experimental imperfections that occurred during the fabrication process, which have been captured in our simulations as we used digitized SEM image as the unit cell. It is important to note that even with the existing fabrication non-idealities, our design performs well as a polarization-independent super absorber. Figure 3: Crossed metallic gratings and broadband, polarization-independent plasmonic super absorbers. ( a ) SEM images of two different crossed metallic gratings with w =60 and 120 nm. Scale bars are 500 nm ( b ) Measured and ( c ) Simulated extinction spectra for two different crossed metallic gratings. ( d ) Extinction spectra for 120-nm-wide crossed-grating structure as a function polarization angle and wavelength. ( e ) SEM image of the fabricated crossed trapezoid arrays (left) and a single unit cell of crossed trapezoid (right). Scale bars are 500 and 100 nm, respectively. ( f ) Measured, and ( g ) Simulated extinction spectra using digitized SEM images (inset) for different incident electric field polarization angles (inset). ( h ) Extinction spectra for crossed trapezoid array as a function polarization angle and wavelength. Full size image We then combined the two approaches identified so far: trapezoid arrays to enable broad spectral extinction and a crossed symmetric arrangement for polarization-independent resonant response. The crossed trapezoid arrays are fabricated using e-beam lithography, and SEM images of such arrays as well as the constituent unit cell are shown in Figure 3e . Measured extinction spectra for two different polarization angles, θ =0° and 45°, are plotted in Figure 3f . For the two different polarization angles, we observed almost identical extinction spectra, confirming that the crossed trapezoid arrays allow for polarization-independent resonant absorption. Moreover, compared with the crossed-grating structures discussed in the previous section, we obtained a much broader and flatter measured extinction peak with a maximum value of 0.9. On average, the measured extinction between 400 and 700 nm is found to be 0.71. To our knowledge, this is the broadest resonant absorption reported for metallo-dielectric absorbers at visible frequencies. We also note that the total thickness of three-layer super absorber structure is only 260 nm, which is clearly a subwavelength over the visible light spectrum range. We simulated the total extinction spectra using digitized SEM images from a 2×2 array (inset Fig. 3g ) for two different polarization angles 0° and 45° as shown in Figure 3g . Again, the measured extinction intensities are lower than that of the simulated extinction due to the difference between light collection method for the experiments and numerical simulations. Simulation predicts an 85% spectral average absorption between 400 and 700 nm with maximum absorption values of 0.99 at 475 nm, 0.98 at 560 nm and 0.95 at 630 nm. Figure 3h plots the polarization angle and wavelength dependence of extinction spectra of crossed trapezoid arrays with 1° angle increments. The overall extinction spectra do not significantly depend on the incident polarization angle. Ideally, the resonant absorption of a black material should not depend on the incident light angle for applications such as blackbody thermal emitters and photovoltaic concentrators. We studied the incidence angle dependence of resonant absorption using full-field electromagnetic simulations. The angle of incidence ( θ i ) ( Fig. 4a ) is varied in 5° steps from 0° to 70° in the simulation. 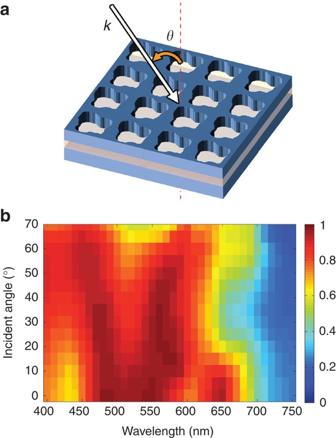Figure 4: Angle of incidence dependence of the resonant extinction. (a) Schematic drawing of a periodic crossed trapezoid arrays with the angle of incidence shown asθ. (b) Extinction plotted as a function of wavelength and angle of incidence. Broadband extinction is preserved even at higher angles of incidence. Figure 4b shows the extinction spectra as a function of wavelength and incident angle. A broadband resonant response is achieved even at high angles of incidence; however, the absorption profile changes slightly with the increased incident angle at certain wavelengths. Below 450 nm, the extinction increases with the increased θ i . This frequency regime is close to the plasma frequency of bulk Ag. At increased angles of incidence, the path length of light in the nanostructures is increasing, thus the light is strongly absorbed at higher angles of incidence. However, around 750 nm, increasing θ i results in decreased extinction. We attribute this angle-dependent absorption at longer wavelengths to Bragg resonances arising from structure periodicity, which are known to be strongly incidence angle dependent. For comparison, we calculated average absorption between 400 and 750 nm for different θ i . At 0°, 5° and 10° the average absorption is around 0.75 and reduces down to 0.70 at 25°. Between 25° and 60°, the average absorption has a constant value around 0.70, and above 60° the absorption reduces by 5% for every 5° steps, down to the value of 0.60 at 70°. Overall, broadband resonant absorption is maintained even at high angles of incidences, a significant achievement for complex nanostructured plasmonic absorbers. Figure 4: Angle of incidence dependence of the resonant extinction. ( a ) Schematic drawing of a periodic crossed trapezoid arrays with the angle of incidence shown as θ . ( b ) Extinction plotted as a function of wavelength and angle of incidence. Broadband extinction is preserved even at higher angles of incidence. Full size image Until now, we have reported the extinction data, which may include light scattered at higher angles that is not collected due to the finite aperture size of the microscope lens in addition to the absorption. Electromagnetic simulation, however, allows us to calculate and compare absorption calculated via different methods. In the simulation, extinction should be approximately equivalent to absorption as the power collected in transmission and reflection monitors placed at the near-field measure the scattered electromagnetic fields as well. Absorption can also be calculated directly, as the power absorbed in any material depends on the divergence of the Poynting vector and may be calculated by the simple relation P abs = 1/2 ω ɛ″| E | 2 for non-magnetic materials, where ω is the frequency, ɛ″ is the imaginary part of the dielectric permittivity and E is the total electric field [16] . 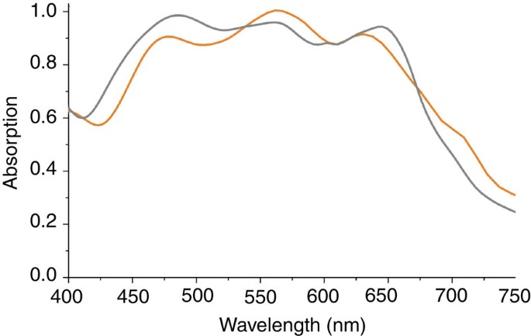Figure 5: Calculated absorption spectra for the broadband plasmonic super absorber. Orange line corresponds to the absorption calculated by theA=1-T-Rformula (same with the 0° data inFig. 3g) and grey line plots the total absorption within the metallic portion of the three-layer MIM stack calculated by using the formulaPabs= 1/2 ω ɛ″|E|2. Electric fields are calculated within a volume monitor, and the resulting absorption spectrum for TE polarization is plotted in Figure 5 . A broadband absorption peak similar to that observed in Figure 3g is achieved, meaning that the extinction is mainly due to the strong light absorption within the metallic sections and the contribution of the scattering to the extinction is negligible. Figure 5: Calculated absorption spectra for the broadband plasmonic super absorber. Orange line corresponds to the absorption calculated by the A =1- T - R formula (same with the 0° data in Fig. 3g ) and grey line plots the total absorption within the metallic portion of the three-layer MIM stack calculated by using the formula P abs = 1/2 ω ɛ″| E | 2 . Full size image Calculating the absorption directly also allows construction of maps of the absorption that enable us to gain more insight into the nature of the absorption processes. 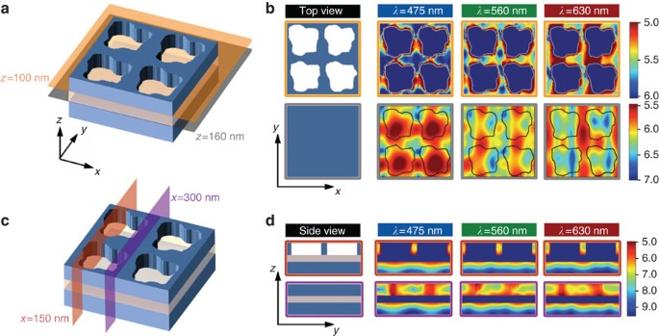Figure 6: Two-dimensional absorption maps displaying absorbed power in metal. (a) Three-dimensional view of simulated absorber structure with cross-sections along the top Ag/SiO2(orange plane) and bottom SiO2/Ag layer (grey plane). (b) Schematic drawing of the metallic section (first column) atz=160 nm (top row) andz=100 nm (bottom row), and corresponding 2D absorption maps at three extinction peak wavelengths, 475 nm (second column), 560 nm (third column) and 630 nm (fourth column). (c)yzcross-sections at two differentxpositions,x=150 nm (red plane) andx=300 nm (purple plane). (d) 2D absorption maps in metallic portion for the indicatedyzplane positions at the peak wavelengths. Graphs inbanddare plotted in logarithmic scale, and red colour corresponds to higher absorption. Figure 6a shows a schematic drawing of the three-dimensional crossed trapezoid array constructed by using the digitized SEM image. The orange and grey planes correspond to the xy planes at two different z values. Power absorbed in the metallic portions at the top Ag/SiO 2 interface at z =160 nm and bottom SiO 2 /Ag interface at z =100 nm are plotted, respectively, in the top and bottom rows of Figure 5b . The right column of Figure 6b displays the metallic cross-section at the given xy plane, whereas the remaining columns plot the power absorbed at the three different peak position wavelengths obtained from Figure 3e : 475, 560 and 630 nm. Note that the absorption maps are plotted using a logarithmic scale, and top and bottom panels have different scales in order to aid visualization of the absorbed power. For this particular simulation, the incident electric field is parallel to the y axis (TE). In the top metal layer, the absorption is stronger around the metal edges due to the higher electric field intensities. Clearly, the absorption is taking place at the different portions of the structured top metal layer. Similarly, for the planar bottom metal layer, we obtained absorption in different sections of the metal at different wavelengths. At 475 nm, power is absorbed at the centre positions corresponding to the air gap of the top metal layer. However, at 560 nm light is absorbed below the narrow section of trapezoid array and at 630 nm absorption is stronger underneath the centre of the trapezoid that is along the y axis. We also calculated absorption in the yz plane at the positions of x =150 nm and x =300 nm, shown in Figure 6c . We observe that power is mainly absorbed on the top-structured Ag layers and within 30 nm of the bottom Ag film ( Fig. 6d ). Figure 6: Two-dimensional absorption maps displaying absorbed power in metal. ( a ) Three-dimensional view of simulated absorber structure with cross-sections along the top Ag/SiO 2 (orange plane) and bottom SiO 2 /Ag layer (grey plane). ( b ) Schematic drawing of the metallic section (first column) at z =160 nm (top row) and z =100 nm (bottom row), and corresponding 2D absorption maps at three extinction peak wavelengths, 475 nm (second column), 560 nm (third column) and 630 nm (fourth column). ( c ) yz cross-sections at two different x positions, x =150 nm (red plane) and x =300 nm (purple plane). ( d ) 2D absorption maps in metallic portion for the indicated yz plane positions at the peak wavelengths. Graphs in b and d are plotted in logarithmic scale, and red colour corresponds to higher absorption. Full size image Plasmonic broadband super absorbers are designed to absorb light in the metallic sections and therefore the absorbed energy is converted to heat. Perfect broadband absorption (unity absorption) could be achieved using multi-layered crossed trapezoid array structures with meticulous control of the dielectric spacers between individual layers. Our design also allows for realization of thin-film thermal emitters and could be used to achieve blackbody emission. Metallic nanostructures with broadband plasmonic resonances proposed in this article are also promising candidates for enhancing the absorption in active semiconductor layers of solar cells over a broad wavelength range. Replacing the dielectric spacer with an active semiconductor with high absorption coefficient could enable broadband absorption and photocarrier generation. Fabrication Quartz glass substrates were first coated with 100 nm thick Ag layers using thermal evaporation. Plasma-enhanced chemical vapour deposition was then utilized to deposit 60 nm thick SiO 2 layers. In order to facilitate pattern transfer by lift-off, we used a bilayer photoresist process. We first spun PMMA 495 A4 at 4,000 r.p.m. and baked it at 180 °C for 2 min. We then spun the second e-beam resist PMMA 950 A2 at 5,000 r.p.m. for 1 min and baked it at 180 °C for 2 min. E-beam lithography was used to define the patterns, and 100 nm Ag layers were deposited on the patterned substrates using thermal evaporation. A lift-off process was performed using acetone, followed by a 2-min ultrasonication process. Optical measurements Optical measurements were performed on an inverted microscope equipped with a spectrometer consisting of a 150-mm focal-length monochromator and liquid-nitrogen-cooled charge-coupled device camera. A broadband halogen lamp was used as a light source and a polarizer was inserted into the light pathway to polarize the incident light. Reflected and transmitted light was collected from 10×10 μ m area using a 50× Zeiss microscope objective with a numerical aperture of 0.55. Transmission was calibrated using a transparent glass substrate. For calibration of reflection, we first measured the reflection from a broadband dielectric mirror (Thorlabs BB2-E02) with an average reflection of 99% between 400 and 850 nm. Measured reflection from nanostructures was then calibrated using the reflection spectra of the dielectric mirrors. Extinction data plotted in this article therefore reflect the total extinction and are not arbitrary. FDTD simulations Full-field electromagnetic wave calculations are performed using Lumerical, a commercially available FDTD simulation software package. A unit cell of the investigated structure is simulated using periodic boundary conditions along the x and y axes, and perfectly matched layers along the propagation of electromagnetic waves ( z axis). Plane waves were launched incident to the unit cell along the + z direction, and reflection is monitored with a power monitor placed behind the radiation source; transmission is monitored with a power monitor placed behind the structure. Electric and magnetic fields are detected within the frequency profile monitors. All of the simulations reported in this paper are performed in three-dimensional layouts. In all of the simulations, we employed cubic mesh with a mesh size of 5 nm. To model Ag in the simulations, we used a Lorentz–Drude formulation from the literature that are tabulated in Rakic's paper [27] , and optical data are plotted in Supplementary Figure S2 . Rakic uses the experimental data from Palik's Handbook of Optical Constants [28] as the experimental data set, and fits to a Lorentz–Drude model for the optical properties. SEM images are digitized using Lumerical's digitization feature. How to cite this article: Aydin, K. et al . Broadband polarization-independent resonant light absorption using ultrathin plasmonic super absorbers. Nat. Commun. x:x doi: 10.1038/ncomms1528 (2011).